Dimensionality of brain networks linked to life-long individual differences in self-control The ability to delay gratification in childhood has been linked to positive outcomes in adolescence and adulthood. Here we examine a subsample of participants from a seminal longitudinal study of self-control throughout a subject’s life span. Self-control, first studied in children at age 4 years, is now re-examined 40 years later, on a task that required control over the contents of working memory. We examine whether patterns of brain activation on this task can reliably distinguish participants with consistently low and high self-control abilities (low versus high delayers). We find that low delayers recruit significantly higher-dimensional neural networks when performing the task compared with high delayers. High delayers are also more homogeneous as a group in their neural patterns compared with low delayers. From these brain patterns, we can predict with 71% accuracy, whether a participant is a high or low delayer. The present results suggest that dimensionality of neural networks is a biological predictor of self-control abilities. The ability to delay gratification as a child has been linked to many important health, social and cognitive outcomes later in life [1] , [2] , [3] , [4] . The neural mechanisms that underlie this association, however, are not understood. The current study draws on a seminal longitudinal examination of self-control over much of the life span, first measured in children at 4 years of age. A subsample of these participants was tested some 40 years later, on a task that required self-control over the contents of working memory. In this study we examined whether patterns of brain activation on this task could distinguish reliably between participants with consistently low and high self-control abilities. One potential driving mechanism for delaying gratification is the ability to keep unwanted or inappropriate information out of working memory so that this information does not unduly influence cognitive processing. For example, the ability to control appetitive impulses that might be in the focus of working memory should help individuals resist immediate temptation on the classic marshmallow test [3] . This delay measure required foregoing an appealing reward, such as a marshmallow, when delaying immediate consumption would lead to increased rewards, two marshmallows. To examine the hypothesis that controlling the contents of working memory is critical to the ability to delay gratification, we capitalized on a unique resource: a group of adults who have a documented life-long history of effective self-control, starting 40 years earlier at age 4 years, and a group of adults who differed from the first group only in having an equally long history of less effective self-control ( Methods and Supplementary Information ). We refer to the former as ‘high delayers’ and the latter as ‘low delayers.’ Therefore, these two samples were quite homogeneous aside from differences in self-control measures across the life span. We examined whether these two groups differ in their neural functioning during a task that requires controlling the contents of working memory by expelling task-irrelevant information. The task was simple: On each trial, six words were presented for storage in working memory, following which participants were directed to forget three of these words. A probe word was then presented, and participants had to indicate whether the probe was one of the remaining stored words. The critical feature of this task is that sometimes participants were presented probe items (‘lures’) that had to be forgotten from working memory; hence, requiring a negative response. Responses to these critical lures were compared with responses to probes that had not been presented in the memory set (‘controls’, that is, probes that were not in memory to begin with; Fig. 1a ). 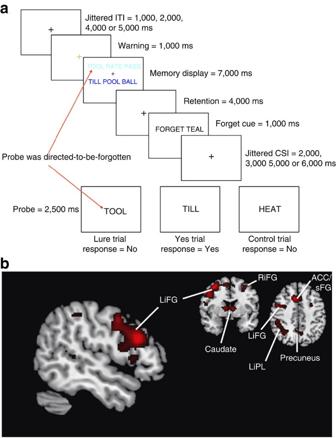Figure 1: Directed-forgetting task and activations. (a) Schematic of the working memory directed-forgetting task. The task is composed of three trial types: lure, yes and control trials. Of most interest is the comparison of accuracy and RT for lure versus control trials. (b) Activation patterns for the lure—control contrast across all participants. Significant activation is seen in the left inferior frontal gyrus (LiFG), the right inferior frontal gyrus (RiFG), the anterior cingulate cortex (ACC)/superior frontral gyrus (sFG), the caudate, the precuneus and the left inferior parietal lobule (LiPL). These images are thresholded atP<0.005 uncorrected for ten contiguous voxels. Figure 1: Directed-forgetting task and activations. ( a ) Schematic of the working memory directed-forgetting task. The task is composed of three trial types: lure, yes and control trials. Of most interest is the comparison of accuracy and RT for lure versus control trials. ( b ) Activation patterns for the lure—control contrast across all participants. Significant activation is seen in the left inferior frontal gyrus (LiFG), the right inferior frontal gyrus (RiFG), the anterior cingulate cortex (ACC)/superior frontral gyrus (sFG), the caudate, the precuneus and the left inferior parietal lobule (LiPL). These images are thresholded at P <0.005 uncorrected for ten contiguous voxels. Full size image If there is a difference between the groups in responses to lure and control trials, it might reveal itself in one or both of two outcomes. First, low-delay participants might have more difficulty responding negatively to lures than high-delay participants revealed as relatively longer response times and relatively poorer accuracy to lure versus control trials. Second, the groups might differ neurally, with low-delay participants exhibiting less efficient neural recruitment during engagement with the working memory task. Dimensionality of neural responses may be an important metric of the efficiency of cortical networks. In longitudinal functional magnetic resonance imaging (fMRI) experiments of stroke recovery, low principal component (PC) dimensionality was found to be related to better post-stroke behavioural recovery [5] . In simulated fMRI data, lower PC dimensionality has been shown to correspond to stronger coupling and/or stronger dynamic range [6] . In other words, intrinsic PC dimensionality is related to the number of distinct strongly covarying networks in fMRI data; if dimensionality is low, then the fMRI signal can be described by a simpler model that contains fewer distinct covarying networks (that is, PCs). Therefore, it is possible that low PC dimensionality may reflect a more efficient recruitment of cortical networks to achieve the same behavioural performance. We define dimensionality by the number of PCs required to optimize classification accuracy between lure and control trials (that is, working memory control). Here we show that low delayers recruited significantly higher-dimensional neural networks when performing the task compared with high delayers. In addition, results indicated that high delayers were more homogeneous as a group in their activation patterns than were low delayers. Finally, utilizing a quadratic discriminant (QD) analysis, we could predict with 71% accuracy whether a participant was a high or a low delayer from their brain activity patterns. The present results suggest that dimensionality of neural networks is a biological predictor of self-control abilities into adulthood. Behavioural results Replicating the standard directed-forgetting effect of slower and less accurate performance on lure trials compared with control trials [7] , [8] , we found a significant main effect of trial type for both reaction time (RT), F (1,22)=58.1, P <0.001 and η p 2 =0.73, and accuracy, F (1,22)=9.6, P <0.01 and η p 2 =0.30. This main effect was present in the low-delay group in RT F (1,11)=47.67, P <0.001 and η p 2 =0.81, and accuracy, F (1,11)=6.71, P <0.05 and η p 2 =0.38, and in the high-delay group in RT, F (1,11)=18.57, P <0.001 and η p 2 =0.63, and a trend in accuracy, F (1,11)=3.62, P =0.08 and η p 2 =0.25. Although there was no interaction between group and trial type for either RT, F (1,22)=0.61, NS, η p 2 =0.03, or ACC, F (1,22)=0.01, NS, η p 2 =0.00, the trends for both measures were in the predicted direction. Specifically, compared with high delayers, low delayers are less accurate and take longer to respond for the lure trials than to the control trials. We also examined differences in lure versus control trials with the combined Z -score of the effects. Again, we found no significant difference between the two groups, t (22)=0.57, NS. We attribute the lack of significance to a small number of experimental trials, high variability in the responses and small overall sample size. Nonetheless, although not reliable in the present experiment, these results hint at the possibility that low-delay participants find it more difficult than do high-delay participants to resolve interference between relevant and irrelevant material in this experiment. More statistical power may be needed to examine whether there is a significant behavioural difference in this task. In addition, there was no main effect of group on either RT, F (1,22)=0.78, NS or ACC, F (1,22)=0.33, NS. Table 1 summarizes the RT and ACC effects by group. Thus, although the difference in response times and accuracy between lure and control trials was numerically greater for the low than for the high delayers, this was not a reliable effect. Table 1 RT and ACC data by group with s.d. in parentheses. Full size table Neural network dimensionality It is important to note that equivalent behavioural performance does not mean that the two groups are resolving interference from lure trials in the same way. Indeed, our neural analyses suggest quite different routes to the same behavioural outcome. What is impressive is that low delayers appear to be recruiting neural networks less efficiently to achieve the same level of behavioural interference control. Linear discriminant (LD) analysis on PCs revealed that low delayers recruited higher-dimensional neural networks than did high delayers when controlling the contents of working memory. In addition, high delayers were more stereotyped in their patterns of brain activation (that is, showed greater homogeneity) than were low delayers, who were characterized by more varied neural networks. On the basis of these findings, we were able to accurately distinguish neural network patterns between high and low delayers with 71% accuracy utilizing a QD analysis. The following three analyses support these conclusions. Dimensionality of individuals’ networks Univariate analyses are limited to treating each voxel in the brain independently, ignoring the spatial patterns and distributions of voxels [9] , and the interactions of different brain locations, all of which have proven important in neuroimaging studies [10] , [11] . To remedy this problem and to examine neural networks, we conducted multivariate analyses using LD analysis on PCs to examine differences in the neural networks recruited for lure and control trials. LD attempts to find a linear combination of voxels that define a plane (that is, each voxel has a weight, and all of the weights together define the plane) that optimally separates two classes of data. This method can be used to classify fMRI volumes according to the task performed during the volume’s acquisition [12] . In addition, the analysis provides a spatial map in which each voxel is assigned a value, indicating the importance of that voxel in the classification [5] . For each participant, 70% of the lure and control trials were used to train the classifier, which was then tested on the remaining 30% of the data to determine classification accuracy [12] ( Methods ). This splitting should provide sufficient data to form a good model, at the same time preserving sufficient data to test the model. In addition, we restricted the analysis to the regions that showed the greatest difference in lure versus control trials ( Fig. 1b ) as uncovered with univariate analyses, a procedure shown to reduce classification errors [13] and to provide an unbiased and orthogonal method from our multivariate analyses to select voxels. This network has been strongly implicated in controlling the contents of working memory [7] , [8] , [14] , [15] and exhibited considerable spatial overlap with previous results ( Supplementary Fig. S1 ), which is why we focused on these associated regions. There was a significant difference between the groups in the number of PCs required to achieve optimal accuracy in classifying trials as lure versus control, t (22)=3.45, P <0.005 and η p 2 =0.35. On average, although 3 PCs were required to optimize classification for high delayers, full 15 PCs were required for low delayers ( Fig. 2 ). This suggests that the network of high delayers is less dimensional and potentially more efficient than is the network of low delayers. 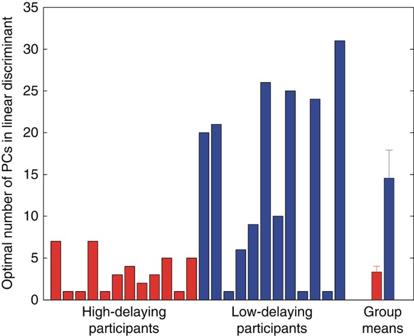Figure 2: The optimal number of dimensions to maximize classification accuracy. The number of LD dimensions/components that were required to achieve maximum classification between lure and control trials for each participant with the group averaged data to the far right. High-delay group=red; low-delay group=blue. Error bars represent s.e.m. Figure 2: The optimal number of dimensions to maximize classification accuracy. The number of LD dimensions/components that were required to achieve maximum classification between lure and control trials for each participant with the group averaged data to the far right. High-delay group=red; low-delay group=blue. Error bars represent s.e.m. Full size image These results were not a function of the splitting proportions between training and test: our results were significant for a 90/10 split, an 80/20 split, a 60/40 split and a 50/50 split ( Table 2 ). In addition, these results were not idiosyncratic to the feature-selected network. When the same analysis was conducted examining all brain voxels (that is, no masking), we obtained the same effect, in which high delayers required fewer PCs than did low delayers to distinguish lure from control trials (6 versus 15), t (22)=2.18, P <0.05 and η p 2 =0.18. Finally, there were no group differences in physiological parameters (heart rate, respiration rate or breath volume), or in the six rigid body motion parameters either at the brain volumes that were analysed or across all brain volumes in the entire functional runs, suggesting that motion and physiology had no role. To control for motion and physiology even further, we covaried motion and physiology ( Methods ) from the raw signal while controlling for the task design. Conducting the analysis on these data yielded the same result of increased dimensionality for the low delayers versus the high delayers (6 versus 14 PCs), t (22)=2.28, P <0.05 and η p 2 =0.19. Therefore, the present findings do not appear to be driven by differences in physiological parameters [16] or motion, nor are the results idiosyncratic to the splitting ratio of the training and test sets or the voxels that were chosen for the analysis. Table 2 Dimensionality differences between the high and low delayers for different proportional splittings of the training and test sets. Full size table Another potential confound in the data was an imbalance in males and females. Our high-delay group contained more females than males (9 out of 12), whereas our low-delay group contained more males than females (8 out of 12). To examine whether gender was a confounding variable in our analysis, we aggregated the data from males and from females to compare the number of PCs to distinguish lure versus control trials (that is, LD dimensionality). This analysis yielded no reliable difference in the number of PCs, t (22)=0.75, NS. Consequently, the dimensionality differences are not driven by gender. Supplementary Figure S2 shows the results of this analysis. Sometimes PC spaces can be difficult to interpret. To allay concerns that our PCs may not be sensible, we plotted the average of the first and second PC separately for each group ( Fig. 3 ), and the first and second PC for each individual participant ( Supplementary Figs S3–S6 ). Examining these plots, and in particular Fig. 3 , the first and second PCs are sensible in that their values are well clustered in our feature-selected network and do not represent disjointed random values spread throughout the space (that is, the values are not salted and peppered throughout the space). Thus, we are confident that the PCs are both plausible and usable. 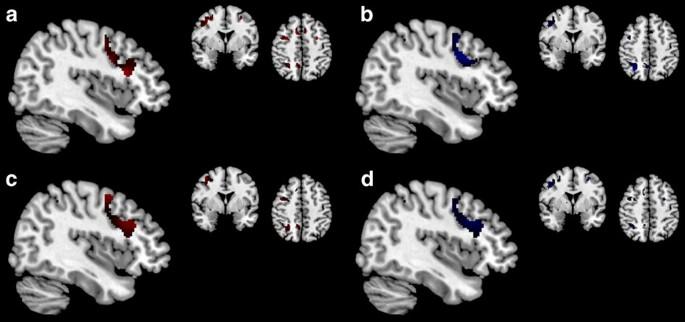Figure 3: Averaged first and second PC for each group. (a) Average PC 1 for high delayers (b) Average PC 1 for low delayers (c) Average PC 2 for high delayers (d) Average PC 2 for low delayers. Figure 3: Averaged first and second PC for each group. ( a ) Average PC 1 for high delayers ( b ) Average PC 1 for low delayers ( c ) Average PC 2 for high delayers ( d ) Average PC 2 for low delayers. Full size image Finally, the same anatomical regions were involved in the classification for both groups: only 16 of the 2,589 voxels showed significant group differences in classification values with univariate t -tests at a liberal threshold of P <0.05, and no voxels surviving a P <0.005 threshold criterion. In sections 2 and 3, we examine these classification maps with multivariate analyses. In sum, this analysis indicates that when controlling the contents of working memory, high delayers activate networks that require fewer dimensions to optimize classification of lure versus control trials than do low delayers, which we posit indicates more efficient neural recruitment. Homogeneity of networks across participants On the basis of the differences in LD dimensionality, we examined differences in homogeneity of the classification maps across the two groups of participants. To evaluate group homogeneity, we measured the Euclidean distance across all voxels from each participant’s LD maps to the mean LD map of all other group members of that participant’s group (either high or low). From this analysis, we could determine how similar or different each participant’s LD classification map was from the mean map of his or her group (excluding that particular participant from the mean map). High delayers had significantly smaller Euclidean distances ( M =0.0022, s.d.=0.0018) than did low delayers ( M =0.0262, s.d.=0.0225), t (22)=3.69, P <0.005 and η p 2 =0.38, suggesting that they are more homogeneous as a group ( Fig. 4 ). 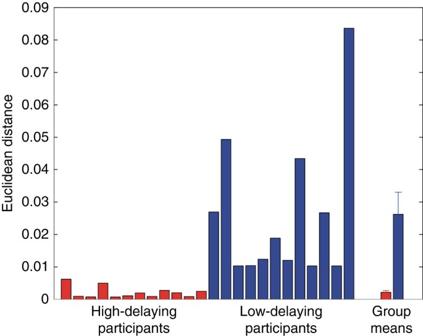Figure 4: The Euclidean distances for each individual participant’s LD map from their group mean LD map. High-delay group=red; low-delay group=blue. Error bars represent s.e.m. Figure 4: The Euclidean distances for each individual participant’s LD map from their group mean LD map. High-delay group=red; low-delay group=blue. Error bars represent s.e.m. Full size image To further examine group homogeneity and to obtain a different visual representation of the data, we performed multi-dimensional scaling (MDS) [17] to plot the first three dimensions of individuals’ LD map values based on the LD map distance matrix (that is, the Euclidean distance of all individual maps from each other as calculated above). In this way, each participant’s entire LD map was summarized by weightings on three dimensions. It is apparent from Fig. 5 that the high-delay group is clustered more tightly, whereas the low-delay group is more heterogeneous. 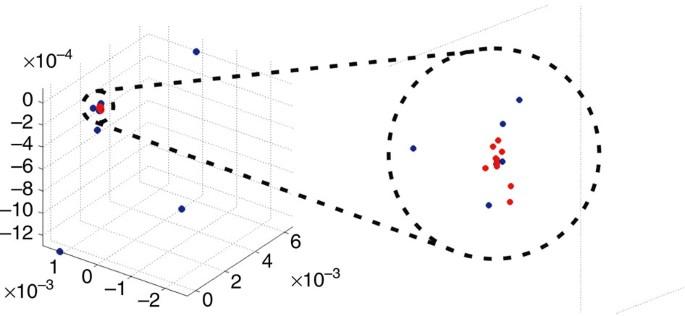Figure 5: MDS results for the first three dimensions of the LD map distance matrix. The high (red) delayers are grouped together more closely than the low delayers (blue). Figure 5: MDS results for the first three dimensions of the LD map distance matrix. The high (red) delayers are grouped together more closely than the low delayers (blue). Full size image Classification of individual participants Examining how the participants were clustered based on our MDS analysis, it was apparent that participants could not be easily classified with a linear decision boundary, though a LD classifier could classify the groups with 58% accuracy, which was above chance. On the basis of the MDS analysis, we classified the groups with a QD, where the decision boundary is a quadratic surface rather than a plane. We implemented a leave-two-out cross-validation framework ( Methods ) and achieved classification accuracy as high as 71.3% (s.d.=0.24%). Using a procedure similar to [12] , we created a sensitivity map that identified the voxels important to the QD classification. Examining the map in Fig. 6 , positive and negative values are distributed across the feature-selected network, particularly in left inferior frontal gyrus, showing that the whole network was involved in classification and that regions were not entirely selective for one group. As a caveat, piecewise interpretations of multivariate maps can be hazardous because of the inclusion of voxel covariances into the analyses, which limits local interpretations; therefore, one should be careful in interpreting the map in Fig. 6 . 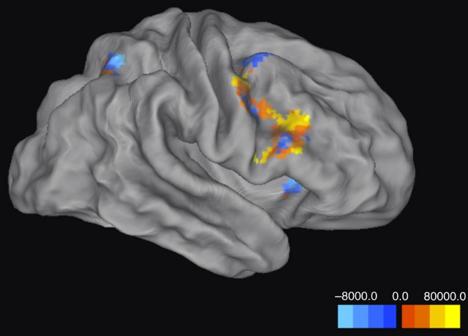Figure 6: QD sensitivity map for classifying high- versus low delayers’ LD maps. Areas in blue represent voxels that are higher in low delayers’ maps. Areas in orange/yellow represent voxels that are higher in high delayers’ maps. The left hemisphere is shown. Figure 6: QD sensitivity map for classifying high- versus low delayers’ LD maps. Areas in blue represent voxels that are higher in low delayers’ maps. Areas in orange/yellow represent voxels that are higher in high delayers’ maps. The left hemisphere is shown. Full size image The QD classifier was a bit more accurate in classifying high delayers than low delayers (73.6 versus 69.0%). This was not surprising given that high delayers were more homogeneous as a group in their pattern of activation and, therefore, clustered together more tightly. Considered collectively, these analyses suggest that dimensionality of brain networks and subsequent classification maps provide important information concerning biological predictors of self-control ability. Univariate fMRI analyses We note that the univariate analyses of these data reveal more commonality than differences between the groups, which may not be surprising given the small behavioural difference in interference between the groups. Across both groups, univariate general linear model analyses revealed significant differences ( Fig. 1b ) for the lure–control contrast in areas such as the left inferior frontal gyrus, the anterior cingulate cortex (ACC) and the left parietal cortex, replicating results from other studies using a similar task [7] , [8] , [14] , [15] and exhibiting considerable spatial overlap with previous results ( Supplementary Fig. S1 ). There were few and modest differences between the low and high delayers in blood-oxygen-level-dependent (BOLD) activation magnitude at liberal thresholds that are summarized in the Supplementary Table S1 . This study demonstrated that self-control ability across the life span is reflected in intrinsic PC dimensionality when performing a task that assesses the ability to control the contents of working memory. Intrinsic PC dimensionality is related to the number of distinct, strongly covarying networks in fMRI data [6] ; for high delayers there are fewer strongly coupled networks to optimize classification of lure versus control trials, and therefore their data can be described by a simpler model that requires fewer PCs. The opposite was true of the low-delay group. Therefore, it is possible that low PC dimensionality reflects a more efficient recruitment of cortical networks for high delayers relative to low delayers to achieve the same behavioural performance on this working memory task. Note that the present findings were obtained in a task that does not challenge participants with information that has emotional or motivational content (as marshmallows do for children or as money might for adults). It may be this lack of affective content that leads to equivalent behavioural performance in high and low delayers on this task; it is possible that with affectively laden stimuli, low delayers would have exhibited a different pattern of behavioural performance in addition to their unique neural signature [18] . Of course, the pattern of neural activations found in the present study must be examined with other cognitive control tasks, but the results offer an important clue for the neural bases of life-long differences in self-control abilities; it is remarkable nonetheless that some 40 years after our participants with well-documented and reliable life-long patterns of high versus low self-control abilities exhibited distinct neural signatures that may represent a biological marker of self-control ability. In this way, the neural dimensionality differences are linked more broadly to behavioural performance—that is, to self-control ability through the life span. Finally, the high-delay group was more homogeneous in their activation patterns than was the low-delay group. This could be interpreted as indicating that life-long self-control is instantiated with more stereotyped neural activation patterns. These findings bring to mind the first line in Leo Tolstoy’s Anna Karenina: ‘All happy families are alike; each unhappy family is unhappy in its own way.’ Perhaps all self-control is alike, but lack of self-control may be instantiated more uniquely. Participants We contacted 117 individuals from more than 500 original participants who completed the delay-of-gratification task at age 4 years at Stanford’s Bing Nursery School during the late 1960s and early 1970s. These 117 individuals were selected because they exhibited either a life-long trajectory of high self-control (above average in their original delay-of-gratification performance, as well as in self-report measures of self-control administered in their 20s and 30s), or a life-long trajectory of low self-regulation (below average on these measures). Of these individuals, 29 participated in this follow-up neuroimaging study and met fMRI safety regulations. Two participants did not complete fMRI scanning, and 3 participants did not complete all 5 runs of the task, leaving us with 24 participants who had complete fMRI imaging data. Please see the Supplementary Information for more details regarding the participants. Directed-forgetting task Participants performed a directed-forgetting working memory task to examine their ability to remove irrelevant information from working memory. Participants saw a display of six words on a screen. Three of the words were presented in blue and three in teal colours. Participants were instructed to encode and remember all six words. After a 4-s delay, participants saw a ‘forget’ cue, indicating the colour of the words they were now to forget; the words in the other colour were to be remembered. Following a jittered cue-to-stimulus interval of 2, 3, 5, or 6 s (average cue-to-stimulus interval=4 s), participants saw a single probe word and pressed a ‘yes’ key if that word was one of the three words they were to remember or a ‘no’ key if it was not one of the three words they were to remember. The intertrial interval was jittered to be 2, 3, 5, or 6 s (average intertrial interval=4 s), which included a 1-s warning display that the next trial was about to begin. Two types of ‘no’ trials were the trials of main interest: those with ‘control’ probes (words that were not seen in over 11 trials on average) and those with ‘lure’ probes (words that were drawn from the to-be-forgotten set of the current trial). Previous research has demonstrated that people are both slower and less accurate in responding to lure trials than to control trials [8] , [14] . The difference in performance between lure and control trials is an index of control over the contents of working memory. There were 100 trials in the task: 50 ‘yes’ trials, 25 ‘lure’ trials and 25 ‘control’ trials. Participants first practiced 20 trials of the directed-forgetting task. All words were of four letters and were taken from previous work [19] . Behavioural analysis parameters A 2 (group: high versus low delay) X 2 (trial type: lure versus control) repeated-measures analysis of variance was conducted on RT (mean RT for correct trials) and accuracy (ACC) data for the ‘no’ trials. The mean RT for correct trials was used in the analysis of RT. Z -scores combining RT and ACC (errors) measures were computed to control for speed/accuracy trade-offs. Classification analysis parameters The de-spiked, smoothed and normalized functional data were mean-centred separately for each run per voxel across time. When constructing within-subject classification maps that distinguished lure versus control trials, the second TR after the onset of the probe stimulus for lure and control trials was analysed. These TRs corresponded to the peak activation of that trial, without having activation bleed into the following trial. In this analysis, all 25 lure trials and 25 control trials were included. We performed feature-selection to select only the voxels that were most active for the lure–control contrast across all participants. This map contained 2,589 voxels that met a threshold of P <0.005 uncorrected at the voxel level for 10 contiguous voxels to reduce and balance type I and type II errors [20] , and also to increase the number of voxels in the feature-selected network (for the subsequent multivariate analyses), because a voxel may not contribute strongly to a univariate effect, but could contribute to a multivariate effect. Data from individual subjects were repeatedly split into training and test sets. The training set was used to train the LD [5] , which was then applied to classify the trials in the test set according to the task performed. The training test was formed by randomly selecting 70% of the trials (with equal number of lure and control trials selected), whereas the remaining 30% formed the test set; we performed 500 such training-test splits. Singular value decomposition [21] was performed on the training data to project it into PC space. Singular value decomposition ranks PCs according to the amount of variance explained. To prevent over-fitting, we used a subset of highest-ranked PCs in our LD analysis, as the lowest-ranked components might contain irrelevant noise specific to the training set. The size of the subset was varied iteratively; we started with only the first PC, then the first 2 PCs and so on, up to the first 34 PCs. At each iteration, test-set data were projected into this PC space, and LD was used to classify the trials into lure and control trials; classification accuracy was recorded. The number of PCs that maximizes classification accuracy serves as our estimate for intrinsic dimensionality of that particular subject’s data. This number of PCs was then used to create LD maps for each individual subject. Motion and physiology covariation To rule out that our dimensionality results were not driven by motion or physiology, we covaried motion and physiology parameters from the raw fMRI signal. We calculated 24 motion parameters, which included the linear, squared, derivative and squared derivative of the six rigid body movement parameters [22] . In addition to these movement parameters, heart rate and two respiratory physiological variables were also added to the analysis. We then mean-centred these parameters and calculated the first PC of these 27 parameters, which we found to account for 90% of the variance in the motion and physiological data. We then regressed this first PC from the mean-centred fMRI signal, as well as regressing out the task design’s convolved hemodynamic response function (HRF) response (which was also mean-centred). We did this because motion and task can be coupled. After performing this regression, we subtracted the beta × the first PC of motion and physiology from the mean-centred fMRI signal and used that signal in the analysis. Leave-two-out cross-validation procedure To examine if individual LD maps could be accurately classified as coming from the high- or low-delay group, the set of 24 LD maps was randomly split into the training set (20 maps, with 10 high and 10 low), the validation set (1 high and 1 low) and the test set (1 high and 1 low). The training set was used to train the LD classifier using a specific number of PCs; this classifier was then used to classify the validation set. The procedure was repeated for different numbers of PCs, from 1 to 19, to determine the number of PCs that optimized classification of the validation set. Finally, the test set was classified using the optimal number of PCs determined on the validation set. This procedure provides an unbiased estimate of classification accuracy of previously unseen (out-of-sample) data. We created 2,000 distinct training-validation-test splits. This same procedure was also conducted when we used the QD classifier instead of the LD classifier. Constructing QD group classification map The spatial map for QD classification was created similarly to the sensitivity map technique described in [5] , with a small but important modification. We computed sensitivity of a voxel as a derivative of the decision function with respect to that voxel, rather than the square of that derivative. By not taking the square, we preserve the sign of the decision function, which encodes the preferred category for that voxel (see also [23] on the sign information in sensitivity maps). Details regarding our fMRI acquisition and pre-processing parameters can be found in the Supplementary Methods . How to cite this article: Berman, M. G. et al. Dimensionality of brain networks linked to life-long individual differences in self-control. Nat. Commun. 4:1373 doi: 10.1038/ncomms2374 (2013).